Points of view in understanding trilobite eyes 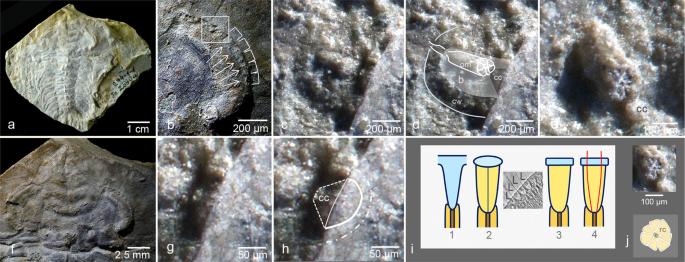Fig. 1: Apposition compound eye and its fossil record. aTrilobiteSchmidtiellus reetaeBergström, 1973, (deposited at the Institute of Geology at Tallinn University of Technology, Estonia, under repository number GIT 294-1., holotype), Lower Cambrian, Estonia, and its compound eye.bAbraded part of the right eye. Note the rectangular sequential elements ‘baskets’ containing the ommatidia.c,d‘Basket’ with ommatidium.eOmmatidium in cross section, showing clearly relics of receptor cells, a central rhabdom and crsytalline cone.fhead ofS. reetae(a).g,hTop part ofc. Crystalline cone and thin cuticle above the ommatidia.iPrinciples of optics in arthropods. 1 Exocone of Xiphosura (Chelicaerata,Limulus), 2 insects, insert: ommatidia of the honey bee (Apis melliferaL.) with a thick, effective cuticular lens in a histological section. Note the crystalline cones below the lenses., 3, 4 crustacean, with ray path in an index gradient lens.jcross-section and schematic drawing of the ommatidium inS. reetae. b ‘basket’, cc crystalline cone, ce cellular wall of the ‘basket’, om ommatidium, L lens, r rhabdom, rc receptor cell; green: lens, pink: crystalline cone, yellow: receptor cell, brown: rhabdom. 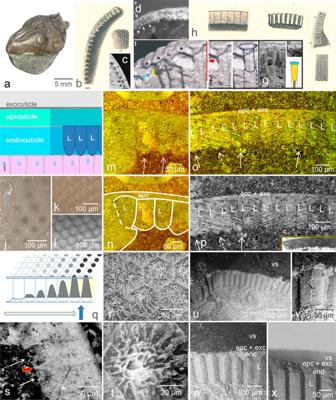Fig. 2: The optical system of asaphid trilobites. aAsaphus(Neoasaphus)expansus(Wahlenberg, 1821), Orthoceras limestone, Ordovician, Sweden [GIK 201].bLindström´s drawing (1901) of lenses hollowed out by decay, continuously weathered from the periphery inwards. Second drawing: View on top of the relics of the lenses, which are filled with dark mud17.c,d[=Fig. 2f, g6] The same specimen, black arrows from Fig. 2f6indicate spine-shaped relics of the weathered prismatic lenses, mistaken in6as crystalline cones (d, bright blue arrow added to Fig. 2f6indicates dividing line between two former lenses).e[=Fig. 3f6]Archegonus wahrsteiniensis, blue arrow and yellow curly bracket, added to the original figure, indicate atypical structure; red curly bracket, added to the original figure Fig. 3f6indicates a section, shown inf.fputative thin lens and crystalline cone, (indicated in blue broken lines, added to the original figure), similar to those ofgDollocaris ingens10.hCylindrical elongated lenses (‘prisms'17) ofA. expansusin the endocuticle, not to be mistaken for crystalline cones, drawn by Lindström17.iSchematic drawing of the structure of the cuticle of arthropods (darkened those parts which can be seen in fossils).jVisual surface ofNileussp. [GIK 202], showing seen from top the phenomenon of mud-filled prismatic lenses, hollowed out by weathering and filled with dark mud.k,IIntact visual surface ofA. raniceps[GIK 203].m,nParabolic to hemicircular refractive inner surfaces of these prismatic lenses [GI R 5011].oSequence of prismatic lenses [GI R 5011].po in black and white to enhance the contrast, making the boundaries between the lenses more visible [GI R 5011].qModel to illustrate, how ‘spines’ and hollow-spaces develop during proceeding weathering [GI R 5011].r,tInitial hollowing out of the lenses seen from the top (Paladin eichwaldi shunnerensis(King 1914)), [GR I 45668].sInitial hollowing out of the lens-prisms (note the arising spine between the arrows) [GI R 5011].uEvidence of elongated lenses in intact visual surfaces ofA. raniceps[GIR 5505], as described by Lindström17. Note the elongated lenses below the exocuticle.vIndividual lens.wSection of the visual surface, showing the exocuticle (dark layer), epicuticle and endocuticular lens prisms. cL cavity of the lens, cv cavity of the crystalline cone, enc endocuticle, epc epicuticle, exc exocuticle, L lens, vs visual surface. [csynchrotron;e,fµ-ct;o–rthin-sections under polarised light;d,j,k,rlight microscope,g,I,s–xSEM. scales:c20 µm,d40 µm,e50 µm,g10 µm. The specimens illustrated here are: Schmidtiellus reetae Bergström, 1973 , Lükati Fm., Atdabanian, Lower Cambrian, Saviranna, Estonia, stored in the collection of the Institute of Geology at Tallinn University of Technology, Estonia, GIT 294-1 [Fig. 1 ]; Asaphus ( Neoasaphus ) expansus (Wahlenberg, 1821), Orthoceras limestone, Ordovician, Sweden, Geologisches Institut der Universität zu Köln, Germany, GIK 201 [Fig. 2a, k, l ]; Asaphus sp., Lindström specimen, Ordovician, Gotska sandön, Gotland, Sweden, Naturhistoriska Riksmuseet, Sektionen för Paleozoologi, Stockholm, Sweden, Ar0059402 [Fig. 2c, d ] [17] ; Archegonus ( Waribole ) warsteinensis (Rud. & E. Richter, 1926), Fammenian, Upper Devonian, Kalvarienberg/Kallenhardt, Germany, Museum für Naturkunde Berlin, Germany, MB.T 7303, [Fig. 2e, f ] [6] ; Dollocaris ingens Van Straelen, 1923, Early Callovian, La Voulte-sur-Rhône Lagerstätte, Middle Jurassic, Ardèche, France, Muséum National d’Histoire Naturelle, Paris, France, MNHN.F.A29278, [Fig. 2g ] [10] . Nileus armadillo (Dalman, 1827), Kunda Fm., Lower Ordovizium, Östergötland/ Schweden, Geologisches Institut der Universität zu Köln, Germany, GIK 202, [Fg. 2j]; Asaphus raniceps Dalman, 1827, Llanvirnian, Lower Ordovician, Haget, northern Oeland, Sweden, Grant Institute of Geology, University of Edinburgh, Scotland, GI R 5011, [Fig. 2m–p, s ]; Paladin eichwaldi shunnerensis (King 1914), Namurian, Mid Carboniferous, Shunner Fell Well, Great Shunner Fell, West Yorkshire, England. GI R 45668 [Fig. 2r, t ]; Asaphus ranicep s Dalman, 1827, lower Llanvirnian, Ordovician, Haget, Öland, Sweden, Grant Institute of Geology, University of Edinburgh, Scotland, GI R 5505, [Fig. 2u–x ]. The specimens here newly documented were photographed with a Keyence digital microscope (VHX-700F, objective VH-Z20T). Reporting summary Further information on research design is available in the Nature Research Reporting Summary linked to this article.